RecurrentCDC25Cmutations drive malignant transformation in FPD/AML Familial platelet disorder (FPD) with predisposition to acute myelogenous leukaemia (AML) is characterized by platelet defects with a propensity for the development of haematological malignancies. Its molecular pathogenesis is poorly understood, except for the role of germline RUNX1 mutations. Here we show that CDC25C mutations are frequently found in FPD/AML patients (53%). Mutated CDC25C disrupts the G2/M checkpoint and promotes cell cycle progression even in the presence of DNA damage, suggesting a critical role for CDC25C in malignant transformation in FPD/AML. The predicted hierarchical architecture shows that CDC25C mutations define a founding pre-leukaemic clone, followed by stepwise acquisition of subclonal mutations that contribute to leukaemia progression. In three of seven individuals with CDC25C mutations, GATA2 is the target of subsequent mutation. Thus, CDC25C is a novel gene target identified in haematological malignancies. CDC25C is also useful as a clinical biomarker that predicts progression of FPD/AML in the early stage. Familial platelet disorder (FPD)/acute myelogenous leukaemia (AML) (MIM601399) is an autosomal dominant disorder with inherited thrombocytopenia, abnormal platelet function and a lifelong risk of the development of a variety of haematological malignancies [1] , such as AML, myelodysplastic syndromes (MDS) and myeloproliferative neoplasms. Although inherited RUNX1 mutations are the cause of the congenital thrombocytopenia, it remains unclear whether a mutation in RUNX1 , which is generally known to have a dominant-negative effect [2] , [3] , [4] , is sufficient to induce the development of haematological malignancies in individuals with FPD/AML. It is also not known whether additional gene mutations are required for the transformation, and, if so, which genes are involved. Given that only 40% of FPD/AML patients develop these neoplasms [5] and that a relatively long period is required for subsequent RUNX1 mutation-mediated development of neoplasms in FPD/AML, the secondary genetic events may function as a driver to promote malignant transformation. We reasoned that identifying gene mutations responsible for the malignant transformation of FPD/AML would provide indispensable information for addressing these questions. However, only about 30 pedigrees with FPD/AML have been reported so far, and the rarity of this disorder has impeded the establishment of clinical diagnostic criteria and the clinical improvement to refine cancer therapy and to identify biomarkers that would allow detection of patients at risk for the onset of malignancies in FPD/AML. We collected DNA samples and clinical information of 73 individuals, belonging to 57 pedigrees, who have a history of familial thrombocytopenia and/or haematological malignancies, with the aim of identifying pedigrees with FPD/AML and uncovering recurrent mutations that drive the malignant transformation. Next-generation sequencing and single-cell sequencing strategy suggest that somatic mutation in CDC25C may be one of the early genetic events for leukaemic initiation in FPD/AML, and further stepwise acquisition of mutations such as GATA2 leads to FPD/AML-associated leukaemic progression. These observations shed light on a part of leukemogenesis in FPD/AML. 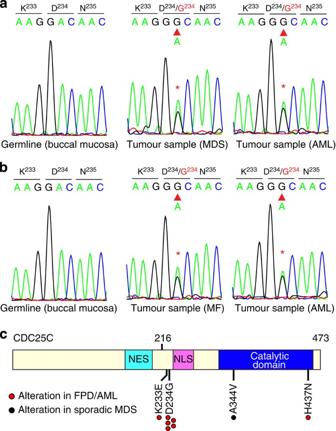Figure 1: Mutation inCDC25Crecurs in cases of FPD/AML. (a,b) Sanger sequencing ofCDC25Cmutations found in whole-exome sequencing is shown. Both forward and reverse traces were available for each mutation, but only one trace is shown above. The results of buccal mucosa, pre-leukaemic phase and leukaemic phase is demonstrated for subject 20 (a) and subject 21 (b), respectively. (c) The distribution of alterations is shown for the CDC25C protein. NES, a putative nuclear export signal domain between amino acids 177–200; NLS, a putative nuclear localization sequence domain consisting of amino acids 240–244. A novel gene target in haematological disorders Thirteen patients in 7 pedigrees were diagnosed as having FPD/AML after screening for germline RUNX1 mutations in 73 index patients; 7 of the 13 patients had developed haematological malignancies, while the other 6 only showed thrombocytopenia ( Table 1 ). Most of the detected RUNX1 mutations were point mutation in Runt homology domain or frame-shift mutation that lost transactivation domain, consistent with the previous reports [2] , [4] . As haploinsufficiency of RUNX1 might cause familial thrombocytopenia with propensity to develop AML [1] , we also examined whether the pedigrees have RUNX1 loss of heterozygosity (LOH) or not. A synchronized quantitative-PCR method [6] and single-nucleotide polymorphism (SNP) sequencing detected no case with LOH in RUNX1 in our cohort ( Supplementary Fig. 1 and detailed in Methods). To systematically identify additional genetic alterations, we utilized whole-exome sequencing for two individuals from the same FPD/AML pedigree who shared a common RUNX1 _p.Phe303fs mutation and who had developed MDS (subject 20) or myelofibrosis (subject 21) at the age of 37 and 17 years, respectively. In both these patients, the disease had progressed to AML [7] . 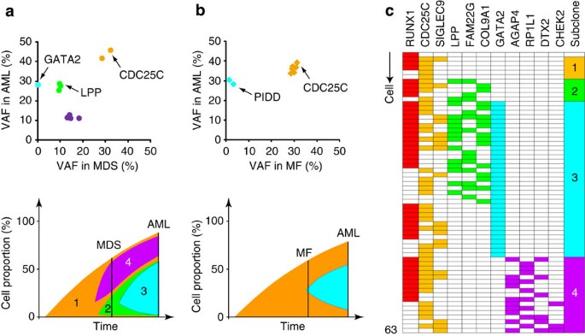Figure 2: Clonal evolution of FPD/AML-related myeloid disorders. (a,b) Observed variant allele fraction (VAF) of validated mutations are listed inTable 2, in both pre-leukaemic and leukaemic phases, are shown in diagonal plots (top) for subject 20 (a) and subject 21 (b). Predicted chronological behaviours in different leukemia subclones are depicted below each diagonal plot. Distinct mutation clusters are displayed by colour. The vertical axis represents cell proportion of each clone calculated by VAF × 2 (%) (because all the mutations were heterozygous), regarding the whole bone marrow as 100%. (c) Mutation status of each bone marrow cell from subject 20 during the acute myeloid leukemia (AML) phase. The vertical axis represents each cell (n=63) and the horizontal axis displays each gene mutation. Coloured columns show that the corresponding cell harbours gene mutation(s) as defined in Online Methods. Subclone numbers shown in the right row correspond to the numbers in the lower figure ofa. Validation by Sanger sequencing and/or targeted deep sequencing of candidate mutations in paired tumour/normal DNA samples confirmed 10 (subject 20) and 8 (subject 21) somatically acquired nonsynonymous mutations ( Table 2 ; Supplementary Figs 2–4 ; Supplementary Methods ). Surprisingly, both patients carried the identical somatic CDC25C mutation (p.Asp234Gly), which had not been reported previously in human cancers ( Fig. 1a,b ). Prompted by this finding, we investigated CDC25C mutations in other FPD/AML cases by deep sequencing. In total, four of seven affected patients with haematological malignancies had CDC25C mutations, of which three carried the same p.Asp234Gly mutation. Moreover, CDC25C mutations were detected in an additional three FPD/AML patients who had not yet developed haematological malignancies, although the variant allele fractions (VAFs) were much lower in this group of patients than in those who had already developed haematological malignancies ( Fig. 1c ; Table 1 ). Thus, 7 of the 13 FPD/AML patients (53%) harboured a CDC25C mutation. CDC25C was also screened for mutations in 90 sporadic MDS and 53 AML patients, including 13 MDS and 3 AML cases who carried RUNX1 mutations. No CDC25C mutations were identified in the 90 sporadic cases, except for the p.Ala344Val in an MDS patient bearing a RUNX1 mutation, indicating that CDC25C mutations were significantly associated with germline, but not with somatic RUNX1 mutations ( P =0.004; Supplementary Fig. 5 ; Supplementary Table 1 ). Table 1 Mutational status of CDC25C in FPD/AML patients. Full size table Table 2 Validated somatic mutations. Full size table Figure 1: Mutation in CDC25C recurs in cases of FPD/AML. ( a , b ) Sanger sequencing of CDC25C mutations found in whole-exome sequencing is shown. Both forward and reverse traces were available for each mutation, but only one trace is shown above. The results of buccal mucosa, pre-leukaemic phase and leukaemic phase is demonstrated for subject 20 ( a ) and subject 21 ( b ), respectively. ( c ) The distribution of alterations is shown for the CDC25C protein. NES, a putative nuclear export signal domain between amino acids 177–200; NLS, a putative nuclear localization sequence domain consisting of amino acids 240–244. Full size image Clonal evolution of FPD/AML Deep sequencing of individual mutations that had been detected by whole-exome sequencing allowed accurate determination of their VAFs; on this basis, we could establish an inferred model of clonal evolution in terms of individual mutations in subjects 20 and 21 ( Fig. 2a,b ; Supplementary Fig. 6a,b ). Intratumoral heterogeneity was evident at both MDS and AML phases in subject 20. According to the predicted model, a founding clone with a CDC25C mutation acquired additional mutations in COL9A1 , FAM22G and LPP (group A), followed by the emergence of a GATA2 mutation (group B), which was associated with leukaemic transformation, whereas the size of another subclone, defined by mutations in CHEK2 and three other genes (group C), was unchanged. To validate this hierarchical model, single-cell genomic sequencing was performed using genomic DNA of 63 bone marrow cells from subject 20 when the patient was in the AML phase. Assuming that all cells harbour the RUNX1 mutation, the false-negative rate of the procedure reached 35%, possibly due to biased allele amplification (Online Methods). However, this technique successfully demonstrated that the group A/B and group C mutations were mutually exclusive ( Fig. 2c ; Supplementary Table 2 ). To statistically evaluate this possibility, we assumed two hypotheses ( H 0 : the mutational status of genes in group A/B and group C is independent; H 1 : mutations in group A/B and group C are mutually exclusive) and calculated each probability distribution ( P i : probability that the current results as shown in Fig. 2c were obtained under the hypothesis H i ). Our mutational profile data were achieved with a much higher likelihood under H 1 than H 0 ( Supplementary Fig. 7 and detailed in Supplementary Methods ). Similarly, the clonal architecture for subject 21 was portrayed in Fig. 2b and Supplementary Fig. 6b . In both scenarios, CDC25C mutations seemed to represent a founding mutation with the highest VAF, suggesting that the CDC25C mutation contributed to the establishment of a founding tumour population as an early genetic event, whereas progression to AML seemed to be accompanied by the appearance of additional mutations, indicating a multistep process in leukemogenesis. Figure 2: Clonal evolution of FPD/AML-related myeloid disorders. ( a , b ) Observed variant allele fraction (VAF) of validated mutations are listed in Table 2 , in both pre-leukaemic and leukaemic phases, are shown in diagonal plots (top) for subject 20 ( a ) and subject 21 ( b ). Predicted chronological behaviours in different leukemia subclones are depicted below each diagonal plot. Distinct mutation clusters are displayed by colour. The vertical axis represents cell proportion of each clone calculated by VAF × 2 (%) (because all the mutations were heterozygous), regarding the whole bone marrow as 100%. ( c ) Mutation status of each bone marrow cell from subject 20 during the acute myeloid leukemia (AML) phase. The vertical axis represents each cell ( n =63) and the horizontal axis displays each gene mutation. Coloured columns show that the corresponding cell harbours gene mutation(s) as defined in Online Methods. Subclone numbers shown in the right row correspond to the numbers in the lower figure of a . Full size image Along with the somatic mutations found in subjects 20 and 21, a GATA2 mutation was also identified in subject 22 ( Fig. 3a ). This patient developed AML with multilineage dysplasia, which led to the diagnosis of AML−MRC (myelodysplasia-related changes). Remission-induction therapies were only partially effective and the blast cell count was reduced from 54 to 5.6%, while dysplastic features persisted ( Fig. 3b ; Supplementary Fig. 8 ). Allogeneic stem cell transplantation was successfully performed from a human leukocyte antigen-matched unrelated donor and durable complete remission, with 100% donor chimerism, was achieved. During treatment, the VAF of the GATA2 mutation decreased virtually in parallel with the blast cell percentage, while the VAF of the CDC25C mutation hovered at a high level before transplantation. Thus, we hypothesized that the GATA2 mutation induced leukaemia progression in this patient, whereas the CDC25C mutation was associated with the pre-leukaemic status. Another GATA2 mutation (p.Leu359Val) was found in subject 18, with a VAF (0.94%), who showed only thrombocytopenia without any signs of leukaemia progression and who had a small subclone with a concurrent CDC25C mutation ( Fig. 3c ). Although GATA2 mutations are detected in a small number of patients with FPD/AML, the findings described above suggest that mutation of GATA2 is a key factor promoting disease progression in FPD/AML ( Fig. 3d ). 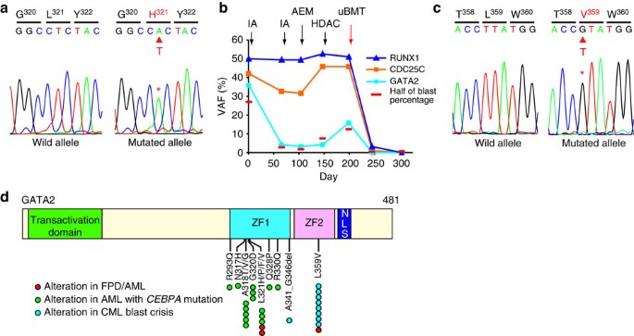Figure 3:GATA2mutations in FPD/AML. The result of Sanger sequencing forGATA2p.Leu321His mutation in subject 22 (a) and Leu359Val mutation in subject 18 (c) validated with subcloning strategy by methods shown inSupplementary Methods. (b) Variant allele fractions (VAFs) ofRUNX1,CDC25CandGATA2mutation in subject 22 are demonstrated with the time course of treatment. Half the value of the blast cell percentage, which corresponds to the allele frequency of a heterozygous mutation, is also shown by a red bar. IA, idarubicine+Ara-C; AEM, Ara-C+etoposide+mitoxantrone; HDAC, high-dose Ara-C; uBMT, unrelated bone marrow transplantation. (d) Schematic representation ofGATA2mutations.GATA2mutations that were identified in FPD/AML are displayed together with mutations found in AML withCEBPAmutation16as well as in CML patients in blast crisis21. ZF, zinc-finger domain; NLS, a putative nuclear localization sequence domain. Figure 3: GATA2 mutations in FPD/AML. The result of Sanger sequencing for GATA2 p.Leu321His mutation in subject 22 ( a ) and Leu359Val mutation in subject 18 ( c ) validated with subcloning strategy by methods shown in Supplementary Methods . ( b ) Variant allele fractions (VAFs) of RUNX1 , CDC25C and GATA2 mutation in subject 22 are demonstrated with the time course of treatment. Half the value of the blast cell percentage, which corresponds to the allele frequency of a heterozygous mutation, is also shown by a red bar. IA, idarubicine+Ara-C; AEM, Ara-C+etoposide+mitoxantrone; HDAC, high-dose Ara-C; uBMT, unrelated bone marrow transplantation. ( d ) Schematic representation of GATA2 mutations. GATA2 mutations that were identified in FPD/AML are displayed together with mutations found in AML with CEBPA mutation [16] as well as in CML patients in blast crisis [21] . ZF, zinc-finger domain; NLS, a putative nuclear localization sequence domain. Full size image Biological consequences of CDC25C mutations We next investigated the possible impact of CDC25C mutation on clonal selection and evolution. CDC25C is a phosphatase that prevents premature mitosis in response to DNA damage at the G2/M checkpoint, while it is constitutively phosphorylated at Ser216 throughout interphase by c-TAK1 (refs 8 , 9 , 10 ). When phosphorylated at Ser216, CDC25C binds to 14-3-3 protein [11] , leading to sequestration of CDC25C to the cytoplasm and its inactivation. Ba/F3 cells were transduced with retroviruses encoding the wild-type or mutant CDC25C containing each of the individual mutations (p.Asp234Gly, p.Ala344Val, p.His437Asn and p.Ser216Ala), and assayed for the phosphorylation status, 14-3-3 protein-binding capacity and intracellular localization of each of these proteins. The Ser216Ala mutant form of CDC25C, which lacks the phosphorylation site, was used as a negative control. In all of the mutated forms of CDC25C, the capacity for binding to c-TAK1 was reduced ( Fig. 4a,b ; Supplementary Fig. 9a,b ), resulting in decreased phosphorylation of CDC25C at Ser216 ( Fig. 4c ). Consequently, the mutant proteins failed to bind 14-3-3 protein efficiently ( Fig. 4d,e ; Supplementary Fig. 8c,d ) and remained in the nucleus even during interphase ( Fig. 4f ; Supplementary Figs 10 and 11 ). In accordance with these observations, CDC25C mutants enhanced mitotic entry, which was exaggerated by low-dose radiation-induced DNA damage ( Fig. 4g,h ; Supplementary Fig. 12 ; Supplementary Methods ). These results suggest that mutation of CDC25C results in disruption of the DNA checkpoint machinery. Next, we investigated why mutation of CDC25C is a frequent genetic event in FPD/AML. It is known that RUNX1 mutations suppress DNA damage repair and subsequent cell cycle arrest in hematopoietic cells by means of transcriptional suppression of several genes that are involved in DNA repair [12] , [13] . We confirmed that FPD/AML-associated RUNX1 mutations have similar effects, as we observed activation of the G2/M checkpoint mechanism in the presence of RUNX1 mutations ( Fig. 4i ; Supplementary Fig. 13a,b ). We found, however, that introduction of mutations in CDC25C resulted in enhanced mitosis entry, despite co-existence of RUNX1 mutations ( Fig. 4i ). Therefore, we speculated that compromised DNA damage checkpoint mechanisms caused by mutations in CDC25C may contribute to malignant transformation, in concert with increased genomic instability due to RUNX1 mutations. 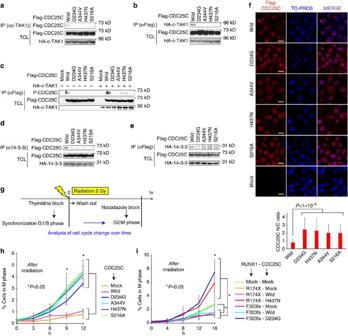Figure 4: Mutated CDC25C enhances mitotic entry. (a) HEK293T cells were transiently transfected with constructs encoding Flag-tagged CDC25C wild type or mutants, as indicated, and cell lysates were immunoprecipitated with anti-c-TAK1 antibody. Binding capacity of CDC25C was evaluated by western blotting. IP, immunoprecipitation; TCL, total cell lysate. (b) Reciprocal immunoprecipitation ofausing anti-Flag (CDC25C) antibody for immunoprecipitation. (c) Left half; cell lysates were immunoprecipitated with anti-Flag antibody. Phosphorylation levels of CDC25C were assessed by phosphorylated-Ser216-specific anti-CDC25C antibody. Right half; the same experiment was performed with cell lysates from HEK293T cells transfected with constructs encoding Flag-tagged CDC25C wild type or mutants and HA-tagged c-TAK1. (d) Mutated CDC25C showed reduced capacity for binding to 14-3-3. Cell lysates were immunoprecipitated with anti-14-3-3 antibody and binding capacity of CDC25C was evaluated. (e) Reciprocal immunoprecipitation ofdusing anti-Flag (CDC25C) antibody for immunoprecipitation. (f) Localization of CDC25C or its mutants was visualized by immunofluorescence. Anti-Flag antibody and Alexa Fluor 555 antibody was used for visualization of CDC25C. N/C ratio of each cell was calculated as detailed inSupplementary MethodsandSupplementary Fig. 10. The mean and s.d. of the N/C ratio is presented. Statistical significance of difference was determined by unpaired Student’st-test (n>30 for each). Scale bar, 10 μm. (g) Schematic description of the method used for evaluation of mitotic entry. (h) Mitotic entry of CDC25C-mutated cells. Percentage of mutated CDC25C-transduced cells in the M phase was compared with that of wild-type CDC25C-transduced cells.Pvalues were calculated using Student’st-test and the differences between groups, as indicated, were all statistically significant (*P<0.05) at 10 and 12 h after irradiation (n=3). The average and s.d. is presented. (i) Mutated RUNX1 and CDC25C were co-expressed in Ba/F3 cells, as indicated, and mitosis entry of these cells was evaluated. The differences between groups, as indicated, were all statistically significant (*P<0.05 at 16 h after washout of thymidine (n=3).Pvalues were determined using the Student’st-test. The average and s.d. is presented. Figure 4: Mutated CDC25C enhances mitotic entry. ( a ) HEK293T cells were transiently transfected with constructs encoding Flag-tagged CDC25C wild type or mutants, as indicated, and cell lysates were immunoprecipitated with anti-c-TAK1 antibody. Binding capacity of CDC25C was evaluated by western blotting. IP, immunoprecipitation; TCL, total cell lysate. ( b ) Reciprocal immunoprecipitation of a using anti-Flag (CDC25C) antibody for immunoprecipitation. ( c ) Left half; cell lysates were immunoprecipitated with anti-Flag antibody. Phosphorylation levels of CDC25C were assessed by phosphorylated-Ser216-specific anti-CDC25C antibody. Right half; the same experiment was performed with cell lysates from HEK293T cells transfected with constructs encoding Flag-tagged CDC25C wild type or mutants and HA-tagged c-TAK1. ( d ) Mutated CDC25C showed reduced capacity for binding to 14-3-3. Cell lysates were immunoprecipitated with anti-14-3-3 antibody and binding capacity of CDC25C was evaluated. ( e ) Reciprocal immunoprecipitation of d using anti-Flag (CDC25C) antibody for immunoprecipitation. ( f ) Localization of CDC25C or its mutants was visualized by immunofluorescence. Anti-Flag antibody and Alexa Fluor 555 antibody was used for visualization of CDC25C. N/C ratio of each cell was calculated as detailed in Supplementary Methods and Supplementary Fig. 10 . The mean and s.d. of the N/C ratio is presented. Statistical significance of difference was determined by unpaired Student’s t- test ( n >30 for each). Scale bar, 10 μm. ( g ) Schematic description of the method used for evaluation of mitotic entry. ( h ) Mitotic entry of CDC25C-mutated cells. Percentage of mutated CDC25C-transduced cells in the M phase was compared with that of wild-type CDC25C-transduced cells. P values were calculated using Student’s t- test and the differences between groups, as indicated, were all statistically significant (* P <0.05) at 10 and 12 h after irradiation ( n =3). The average and s.d. is presented. ( i ) Mutated RUNX1 and CDC25C were co-expressed in Ba/F3 cells, as indicated, and mitosis entry of these cells was evaluated. The differences between groups, as indicated, were all statistically significant (* P <0.05 at 16 h after washout of thymidine ( n =3). P values were determined using the Student’s t- test. The average and s.d. is presented. Full size image Whole-exome sequencing, followed by targeted deep sequencing, identified novel aspects of the pathogenesis of malignant transformation in FPD/AML. First, the high frequency of CDC25C mutations in FPD/AML underscores their major role in the development of haematological malignancies in FPD/AML patients. To our knowledge, CDC25C mutations have not been reported previously and represent a new recurrent mutational target in haematological malignancies, although CDC25C mutations have been reported in some solid carcinomas with unknown significance [14] , [15] . Furthermore, our functional assays support their biological significance, which is characterized by cell cycle progression and premature mitotic entry. Although the 5q31 minimally deleted region, in which CDC25C is located, is frequently detected in MDS, it seems to be associated with other oncogenic mechanisms since our functional assays suggested that CDC25C mutations in FPD/AML were gain-of-function type mutations that facilitate the mitotic entry by aberrant accumulation in the nucleus. Impaired DNA repair function mediated by germline RUNX1 mutation may play a role in the generation of CDC25C mutations. Evaluation of the allelic burden of mutated genes demonstrated that CDC25 mutations are found with high VAFs in FPD/AML-derived leukaemia and with low VAFs in cases of thrombocytopenia. Our hierarchical model and clonal selection highlighted that mutation of CDC25C defines an initial event during malignant transformation and predates subclonal mutations in GATA2 and other genes. On the basis of the observation that four of the seven FPD/AML patients with CDC25C mutations have developed leukaemia and that CDC25C mutations were actually detected in the leukaemic subclones, we speculated that a FPD/AML patient with a CDC25C mutation, but without clinically evident leukaemia, is at high risk for the onset of leukaemic progression. Examination of the allelic burden of CDC25C mutation may thus serve to evaluate the risk of leukaemic progression in patients with FPD/AML. Among the mutations found in FPD/AML, mutations in GATA2 were identified in 3 of 13 individuals (subjects 18, 20 and 22). GATA2 mutations were frequently identified in FPD/AML-derived leukaemia (2/7) and in a patient with thrombocytopenia who had a small subclone bearing a CDC25C mutation (1/6). Although reports on the clinical relevance of GATA2 mutations in myeloid malignancy are limited, several lines of evidence in this respect have recently been reported. GATA2 mutations are frequently found in a subgroup of patients with cytogenetically normal AML with biallelic CEBPA gene mutations [16] , which account for ~4% of AML. Germline GATA2 mutations are also observed in disorders linked to an increased propensity for the development of MDS and AML, including Emberger syndrome, MonoMAC syndrome and dendritic cells, monocytes, B and natural killer cells deficiency [17] , [18] , [19] , [20] . The alterations in GATA2 (leading to p.Leu321His and p.Leu359Val), which were found in FPD/AML patients in this study, are located in the part of the gene encoding the N-terminal and C-terminal zinc-finger domains, respectively ( Fig. 3d ). Mutations affecting the identical amino acids have been reported in AML patients bearing CEBPA mutations and chronic myeloid leukaemia patients in blast crisis [16] , [21] . Thus, GATA2 mutation may contribute to AML progression in collaboration with RUNX1 and/or CDC25C mutations. Furthermore, although another report identified somatic CBL mutation with acquired 11q uniparental disomy as a second hit as being responsible for leukaemic transformation in FPD/AML [22] , CBL mutations were not detected in our series of FPD/AML samples. Although the precise pathogenetic roles of CDC25C mutations remain unclear, we presume that mutant CDC25C alleles confer a proliferative advantage under certain circumstances in which DNA repair machinery is compromised, such as that mediated by a germline RUNX1 mutation. In addition, as Turowski and colleagues reported that CDC25C was involved in S phase entry in addition to mitotic entry [23] , release from thymidine-induced G1/S block may be affected by some unknown machinery mediated by mutated CDC25Cs, which might affect the results when we observed G2/M phase fraction of these cells. It is not clear why CDC25C mutations are repetitively documented in FPD/AML, but not in sporadic MDS or AML cases. One possibility is that in the presence of a RUNX1 mutation, as an initial event, an extended period is required before an additional CDC25C mutation is acquired. This proposal is supported by the clinical observation that ~40% of patients with FPD/AML develop leukaemia in their 30s [5] ; however, the mutational status in CDC25C in the reported cohort was unknown. One of the important problems in the research of FPD/AML is that definitive diagnostic criteria have not been established yet. For this purpose, more extensive studies are required for accumulating clinical characterization, genetic information and functional examination as to whether a RUNX1 variant in families with thrombocytopenia and/or haematological malignancy is causal [24] . We clarified tentative diagnostic criteria for FPD/AML, which was used in this study (in Methods). Regarding the three missense variants in our study (p.Ser140Asn in pedigree 54, p.Gly172Glu in pedigree 57 and p.Leu445Pro in pedigree 32), Ser140 and Gly172 have been reported to be mutated in sporadic AML and/or MDS cases [25] , [26] . In addition, induced pluripotent stem cells from a FPD/AML pedigree with p.Gly172Glu recapitulate the phenotype of FPD/AML after hematopoietic differentiation [27] . Ser140 has been also shown to be important for RUNX1 conformation, and a mutation of this site affects hydrogen bonds and results in functional loss [28] , [29] . Furthermore, all the three missense variants have not been reported in the following SNP database: SNP database (dbSNP) ( http://www.ncbi.nlm.nih.gov/projects/SNP ), the 1000 Genomes Project ( http://www.1000genomes.org ), HGVB ( http://www.genome.med.kyoto-u.ac.jp/SnpDB/index.html ). They were also predicted as ‘damaging’ by Polyphen-2 ( http://genetics.bwh.harvard.edu/pph2/ ), SIFT ( http://sift.jcvi.org/ ) and PROVEAN ( http://provean.jcvi.org/index.php ). Therefore, we regarded the pedigrees with these RUNX1 variants as having FPD/AML in this study. However, regarding pedigree 32 with p.Leu445Pro, we could not completely exclude the possibility of incidental co-occurrence of a possible non-causal RUNX1 germline variant and hairy cell leukaemia, although co-occurrence of them is supposed to be rare. In addition, we should bear in mind the somatic as well as germline LOH of RUNX1 , which contributes to thrombocytopenia and/or leukemogenesis in FPD/AML. In conclusion, our results indicate that FPD/AML-associated leukaemic transformation is due to stepwise acquisition of mutations and clonal selection, which is initiated by a CDC25C mutation in the pre-leukaemic phase, and is further driven by mutations in other genes including GATA2 ( Supplementary Fig. 14 ). The identification of CDC25C as the target gene responsible for the leukaemic transformation will facilitate diagnosis and monitoring of individuals with FPD/AML, who are at an increased risk of developing life-threatening haematological malignancy. Subjects Studies involving human subjects were done in accordance with the ethical guidelines for biomedical research involving human subjects, which was developed by the Ministry of Health, Labour and Welfare, Japan; the Ministry of Education, Culture, Sports, Science, and Technology, Japan; and the Ministry of Economy, Trade, and Industry, Japan, and enforced on 29 March 2001. This study was approved by ethical committee of the University of Tokyo and each participating institution. Written informed consent was obtained from all patients whose samples were collected after the guideline was enforced. All animal experiments were approved by the University of Tokyo Ethics Committee for Animal Experiments. The clinical data, peripheral blood sample and buccal mucosa of the patients whose pedigree contained two or more individuals with thrombocytopenia and/or any haematological malignancies were collected from participating institutions. Platelet threshold depended on each institution’s judge and any haematological malignancies were allowed. The diagnoses were self-reported. When all the following four criteria were fulfilled, the patient was considered as having FPD/AML in this study: (1) the pedigree has two or more individuals with thrombocytopenia and/or any haematological malignancies; (2) a germline RUNX1 variant, including missense, nonsense, frameshift, insertion and deletion, is confirmed by Sanger sequencing and a synchronized quantitative-PCR method in at least one family member; (3) the RUNX1 variant has not been reported in public dbSNP; (4) no germline mutations were detected in the following 16 genes: GATA2 , GATA1 , CEBPA , MPL , MYH9 , MYL9 , GP1BA , GP9 , MASTL , HOXA11 , CBL , DIDO1 , TERT , ANKRD26 , GFI1B and SRP72 . Regarding the last criterion, 16 genes were selected because they have been reported to be responsible for familial thrombocytopenia and/or haematological malignancies. Whole-exome sequencing Genomic DNA was extracted from samples using the QIAamp DNA Mini kit (Qiagen). Exome capture was performed. Enriched exome fragments were subjected to sequencing using HiSeq2000 (Illumina). We removed any potential somatic mutations that were observed in dbSNP ( http://www.ncbi.nlm.nih.gov/projects/SNP ) or in the 1000 Genomes Project ( http://www.1000genomes.org ) data. All candidate single-nucleotide variations and indels, which were predicted to be deleterious by the Polyphen-2 algorithm, were validated by deep sequencing and Sanger sequencing. Genomic DNA samples from the buccal mucosa of the two patients (subject 20 and subject 21) were used as references. All candidate somatic mutations were validated by Sanger sequence and deep sequencing using primers listed in Supplementary Tables 3 and 4 . Deep sequencing Using genomic DNA of the patients as template, each targeted region was PCR amplified with specific primers ( Supplementary Table 4 ). The amplification products from an individual sample were combined and purified with the AMpure XP Kit (Beckman Coulter) and library preparation was carried out using the Ion Xpress Fragment Library Kit (Life Technologies) according to the manufacturer’s instructions. The Agilent 2100 Bioanalyzer (Agilent Technologies) and the associated High Sensitivity DNA kit (Agilent Technologies) were used to determine quality and concentration of the libraries. The amount of the library required for template preparation was calculated using the template dilution factor calculation described in the protocol. Emulsion PCR and enrichment steps were carried out using the Ion OneTouch 200 Template Kit v2 DL (Life Technologies). Sequencing was undertaken using Ion Torrent PGM and Ion 318 chips Kit v2 (Life Technologies). The Ion PGM 200 Sequencing Kit (Life Technologies) was used for sequencing reactions, following the recommended protocol. The presence of CDC25C and GATA2 mutations was also validated by a subclone strategy for DNA sequence analysis. Single-cell sequencing and genome amplification Single cells were separated from the bone marrow of subject 20 at AML phase using FACSAria II (BD biosciences) ( Supplementary Fig. 15a ). Each cell was deposited into individual wells of a 96-well plate. Single cells were lysed and whole genome from single cell was amplified using GenomePlex Single Cell Whole-Genome Amplification Kit (Sigma-Aldrich). Mutation status of each gene was analysed by direct sequencing with specific primers ( Supplementary Table 5 ). To improve the sensitivity of this procedure, we used multiple primer sets for detecting a single-nucleotide variation. We estimated the false-negative rate of this procedure based on the ratio of RUNX1 mutation, which is supposed to be observed in all of the cells. The false-negative rate was estimated to be 35% (22 cells out of 63 cells, Supplementary Table 2 ), which is consistent with the manufacturer’s bulletin reporting the allelic dropout of 30%. In light of these results, we regard those cells with at least one gene mutation in a mutational group (coloured in red, orange, green, blue or purple) as being positive for gene mutations of the corresponding group. To assess whether mutations in LPP , FAM22G , COL9A1 and GATA2 and mutations in AGAP4 , RP1L1 , DTX2 and CHEK2 were mutually exclusive, we performed a statistical analysis as follows. First of all, we determine a matrix A that virtually represents the mutational status of eight genes (1: LPP , 2: FAM22G , 3: COL9A1 , 4: GATA2 , 5: AGAP4 , 6: RP1L1 , 7: DTX2 and 8: CHEK2 ) of 57 cells. Concretely, A is defined as follows: On the other hand, a matrix R indicates data from the actual experimental results of mutational analysis as shown in Fig. 2c . Elements of R is provided in Supplementary Table 2 . Then we assumed two hypotheses: H 0 and H 1 . H 0 : the mutational status of genes 1~4 and genes 5~8 is independent. Each matrix elements of A are randomly assigned 0 or 1 (at ratio of 1:1) independently of each other. H 1 : mutations in genes 1~4 and genes 5~8 are mutually exclusive, and cells 1~40 harbour mutations of genes 1~4, while cells 41~57 harbour mutations of genes 5~8. In mathematical representation, We assumed matrices A 0 and A 1 that represent virtually generated mutational status under the hypotheses H 0 and H 1 , and calculate the probability of substantializing R for given A 0 and A 1 . P 0 ( R / A 0 ) and P 1 ( R / A 1 ) can be calculated for given matrices A 0 and A 1 under the condition as follows: Probability that we cannot determine whether a cell has mutation in gene X when the cell does not actually have a mutation; 28% (based on our data shown in Supplementary Table 2 ). Probability that we judge that a cell has a mutation in gene X when the cell does not actually have a mutation; 5% (because it is very unlikely to happen). Probability that we can judge correctly that a cell does not have a mutation in gene X when the cell does not actually have a mutation; 67% (100−28−5=67%). Probability that we cannot determine whether a cell has mutation in gene X when the cell actually has a mutation; 28% (based on our data shown in Supplementary Table 2 ). Probability that we judge that a cell has a mutation in gene X when the cell actually has a mutation; 35% (the estimated false-negative rate based on the ratio of RUNX1 mutation). Probability that we can judge correctly that a cell has a mutation in gene X when the cell actually has a mutation; 37% (100−28−35=37%). Put it simply, P 0 represents the probability that one can get the mutational profile R when a cell harbours mutations independently of each other, while P 1 indicates the probability that R is realized under the condition where mutations in gene groups 1~4 and 5~8 are exclusive. Because A 0 and A 1 that meet the hypotheses H 0 and H 1 can be generated innumerably, we conducted a computational simulation to acquire the distribution of P 0 and P 1 by generating A 0 and A 1 100,000 times. For visibility, horizontal axis is converted to −In( P ). Synchronized quantitative-PCR These experiments were performed mostly as described previously [6] . Briefly, genomic DNA was denatured 95 °C for 5 min and iced immediately. Using the LightCycler 480 Instrument II (Roche), thermal cycling was performed with denatured genomic DNA, forward and reverse primers ( Supplementary Table 6 ), THUNDERBIRD SYBR qPCR mix (TOYOBO). Threshold cycle scores were determined as the average of triplicate samples. We designed 27 primers for RUNX1 and 3 reproducible primers (that is, primer RUNX-9, RUNX-19 and RUNX-20) were chosen by preparatory experiments. RPL5-2 and PRS7-1 primers, which were authorized previously [6] , were also utilized as controls. In addition, genomic DNA extracted from the bone marrow sample of a MDS patient with a chromosome 21 deletion was also examined with the same primers as a control of RUNX1 locus copy-number loss. Crossing points (Cps) of designed primers were examined by quantitative PCR. RUNX1 locus copy-number relative to RPL5-2 was calculated using Cps of RUNX-9 and RPL5-2, with RPL5-2 values set at 2. Similar results were obtained when Cps of RUNX-19, RUNX-20 or RPS7-1 values were used. LOH detection with SNP sequencing To examine the existence of uniparental disomy, we designed four specific primers to detect nine SNPs in RUNX1 , which are frequently seen (>40%) ( Supplementary Table 7 ). Direct sequencing was performed with the primers, and heterogeneity of SNPs was examined. Chemicals and immunological reagents Thymidine and nocodazole were purchased from Sigma-Aldrich. Anti-CDC25C, anti-phospho-CDC25C (Ser216) and anti-beta-actin antibodies were purchased from Cell Signaling Technology. Anti-HA monoclonal antibody was purchased from MBL. Rabbit anti-Flag monoclonal antibody was purchased from Sigma-Aldrich. Anti-HA was purchased from Roche. Mouse anti-phospho-histone H2AX (Ser139) antibody and Alexa Fluor 488 mouse anti-phospho-H3 (Ser10) antibody were purchased from Merck Millipore. Alexa Fluor 488 rabbit anti-mouse immunoglobulin (Ig)G, Alexa Fluor 488 goat anti-rabbit IgG and Alexa Fluor 555 goat anti-rabbit IgG were purchased from Invitrogen. TO-PRO3 was purchased from Molecular Probes. Rabbit anti-14-3-3 Sigma antibody was purchased from Bethyl laboratories. Sheep anti-c-TAK1 antibody was purchased from Exalpha Biologicals. Anti-sheep IgG-HRP was purchased from RSD. Nonviable cell exclusion was performed by 7-AAD Viability Staining Solution (BioLegend). Subclone strategy and direct sequencing Using genomic DNA of the patients as template, each targeted region was amplified by PCR with specific primers ( Supplementary Table 4 ). PCR products were purified with illustra ExoStar (GE Healthcare) and subcloned into Eco RV site of pBluescript II KS(−) (Stratagene). Ligated plasmids were transformed into E. coli strain XL1-Blue by 45 s heat shock at 42 °C. Positive transformants were incubated on LB plates containing 100 μg ml −1 ampicillin supplemented with X-gal (Sigma-Aldrich) and isopropyl β-D-1-thiogalactopyranoside (Sigma-Aldrich). For colony PCR, a portion of a white colony was directly added to a PCR mixture as the DNA template. Insert region was amplified by PCR procedure with T3 and T7 universal primers, purified with illustra ExoStar (GE Healthcare Life Sciences), and sequenced by the Sanger method with T3 and T7 primers using BigDye Terminator v3.1 Cycle Sequencing kit (Applied Biosystems) and ABI Prism 310 Genetic Analyzer (Life Technologies). Immunoprecipitation and western blotting These experiments were performed as described previously [30] . Briefly, HEK293T cells were transiently transfected with mammalian expression plasmids encoding Flag-tagged CDC25C and its mutants, HA-tagged 14-3-3 or c-TAK1. All plasmids were sequence verified. After 48 h, cell lysates were collected and incubated with an antibody (anti-HA antibody (1:200, 3 h), anti-Flag antibody (1:200, 3 h), anti-c-TAK1 antibody (1:150, 3 h) and anti 14-3-3 antibody (1:150, 3 h)). After incubation, the cell lysates were incubated with protein G-Sepharose (GE Healthcare) for 1 h. The precipitates were stringently washed with high salt-containing wash buffer and analysed by western blotting. Anti-Flag (HRP-conjugated, Sigma-Aldrich), anti-HA (MBL), anti-HA (HRP-conjugated, Roche), anti-CDC25C (Cell Signaling Technology), anti-phospho-CDC25C (Ser216) (Cell Signaling Technology), anti-c-TAK1 antibody (Exalpha Biologicals) or anti-14-3-3 antibody (Bethyl laboratories) antibodies and Immunostar LD (Wako) was used for detection. Original gel images of western blot analysis are shown in Supplementary Fig. 16 . Cell cycle synchronization and analysis for mitosis entry After transduction of wild-type CDC25C or its mutated forms to murine lymphoid cell line Ba/F3 cells (RIKEN BioResource Center), double-thymidine block was performed to obtain cell cycle synchronization at G1/S phase. In brief, 2 mM of thymidine was added to the medium. After 16 h, cells were washed and released from the first thymidine for 8 h. A second block was initiated by adding 2 mM of thymidine, and cells were maintained for 16 h. Then thymidine was washed out and the cells were incubated with 1 mM nocodazole with or without 2 Gy of irradiation ( Supplementary Fig. 10a ). Ba/F3 cells were fixed over time with 75% ethanol in phosphate-buffered saline (PBS) at 4 °C overnight and permeabilized with 2% Triton-X at 4 °C for 15 min. The cells were stained with anti-phospho-H3 (Ser10) Alexa Fluor 488 conjugated antibody (dilution, 1:200) in PBS with 2% fetal calf serum at 4 °C for 30 min and then treated with 5% propidium iodide and 1% RNase in PBS at room temperature (RT) for 30 min. Cell cycle was analysed using a BD LSR II Flow cytometer (BD biosciences) ( Supplementary Fig. 15b ). To assess the cooperation of CDC25C and RUNX1 mutation, wild-type or mutant (D234G, H437N) pMXs-neo-Flag-CDC25C and mutant (F303fsX566, R174X) pGCDNsam-IRES-KusabiraOrange-Flag-RUNX1 were retrovirally transduced into Ba/F3 cells. Immunofluorescent microscopic analysis These experiments were performed as described previously [30] . Briefly, Ba/F3 cells were fixed, permeabilized and blocked. Staining for phosphorylated histone H2AX was performed with anti-phospho-histone H2AX (Ser139) antibody (dilution, 1:500; Merck Millipore) at RT for 3 h. After washing with PBS three times and with 1% bovine serum albumin in PBS, the cells were treated with Alexa Fluor 488 rabbit anti-mouse IgG (dilution, 1:500; Invitrogen) and TO-PRO3 (dilution, 1:1,000; Molecular Probes) for 1 h. The proteins were visualized using FV10i (Olympus) or BZ-9000 (Keyence). The percentage of γH2AX foci-positive cells was determined by examining 100 cells per sample. Three independent experiments were performed. To evaluate the localization of CDC25C, Ba/F3 cells were treated with 2 mM thymidine for 12 h and stained. Staining was underwent with anti-Flag antibody or anti-CDC25C antibody at RT for 3 h. After washing, the cells were treated with Alexa Fluor 488 or 555 antibody and TO-PRO3 for 1 h. The mean intensity of CDC25C in the nucleus and cytoplasm of each cell was measured within a region of interest placed within the nucleus and cytoplasm ( Supplementary Fig. 10 ). Similarly, the background intensity was quantified within the region of interest placed outside the cells. All the measurements were performed using the Fluoview FV10i software or ImageJ. The background-subtracted intensity ratio of the nucleus to cytoplasm was calculated in >30 cells in each specimen. Retrovirus production The procedures were performed as described previously [30] . Briefly, Plat-E packaging cells were transiently transfected with each retroviral construct using the calcium phosphate precipitation method, and supernatant containing retrovirus was collected 48 h after transfection and used for infection after it was centrifuged overnight at 10,000 r.p.m. Statistical analysis To compare data between groups, unpaired Student’s t- test was used when equal variance were met by the F -test. When unequal variances were detected, the Welch t- test was used. Differences were considered statistically significant at a P value of <0.05. Accession codes: Sequence data for FPD/AML patients has been deposited in GenBank/EMBL/DDBJ sequence read archive (SRA) under the accession code SRP043031 How to cite this article : Yoshimi, A. et al. Recurrent CDC25C mutations drive malignant transformation in FPD/AML. Nat. Commun. 5:4770 doi: 10.1038/ncomms5770 (2014).